Three-dimensional analysis of Nafion layers in fuel cell electrodes Proton exchange membrane fuel cell is one of the most promising zero-emission power sources for automotive or stationary applications. However, their cost and lifetime remain the two major key issues for a widespread commercialization. Consequently, much attention has been devoted to optimizing the membrane/electrode assembly that constitute the fuel cell core. The electrodes consist of carbon black supporting Pt nanoparticles and Nafion as the ionomer binder. Although the ionomer plays a crucial role as ionic conductor through the electrode, little is known about its distribution inside the electrode. Here we report the three-dimensional morphology of the Nafion thin layer surrounding the carbon particles, which is imaged using electron tomography. The analyses reveal that doubling the amount of Nafion in the electrode leads to a twofold increase in its degree of coverage of the carbon, while the thickness of the layer, around 7 nm, is unchanged. The development of alternative energies is a critical issue because of the increasing scarcity of fossil fuels and the pollution problems associated with their use [1] , [2] . In this regard, proton exchange membrane fuel cells (PEMFCs) are recognized as one of the most promising energy-converting devices to obtain electrical energy through electrochemical reactions without generation of pollutants [3] , [4] . The membrane electrode assembly (MEA) is the key component influencing the performance, the long-term stability and the production costs of a PEMFC. It is composed of a proton-conducting membrane coated on each side with electrodes involving a catalyst layer where the electrochemical reactions take place. The catalyst layer itself is a composite porous nanomaterial generally consisting of carbon black (CB) supporting platinum nanoparticles (the catalyst) and using an ionomer as both binder and electrolyte [4] , [5] , [6] . Reference materials for the proton exchange membrane and for the ionomer in the catalyst layer are perfluorosulfonated ionomers, whose most famous example is commercialized under the trade name Nafion. In the electrodes, the electrochemical performance can be limited by the transport of protons, electrons or reactant gases (H 2 and O 2 ) to the catalyst sites. Consequently, the MEA multiscale microstructure strongly influences the performance of a PEMFC [7] , [8] , [9] . Much research work has been devoted to enhance the microstructure in the cathode electrode in order to optimize the degree of Pt utilization under operation that is estimated to be of ~10–20% in state-of-the-art electrodes [10] . This optimization is necessary to reduce the Pt loading and therefore the cost of a PEMFC. The structure of the ionomer network inside the active layer is probably the main factor that affects the degree of Pt utilization. Indeed, this must ensure both ionic contact with a maximum of Pt nanoparticles and the connectivity of the ionic conduction paths to the membrane without inhibiting the gas diffusivity. Despite the crucial role of the ionomer layer, there exist presently very few experimental data on the ionomer distribution within the electrode. Hitchcock and co-workers [11] demonstrated the capabilities of synchrotron soft X-ray microscopy tomography method for mapping in 3D the ionomer across the electrode; however, at a more local length scale, the currently only available information about the morphology of the Nafion layer surrounding the CB is the thickness, which was estimated to be ~5–10 nm from selected transmission electron microscopy (TEM) images [12] , [13] . The present work shows for the first time a 3D characterization of this Nafion layer at the nanometre scale. 3D reconstructions obtained by electron tomography can indeed provide critical parameters for understanding and improving such structures, for example, the thickness and the degree of coverage of the CB particles by the ionomer. Electron tomography Electron tomography performed in a high-angle annular dark-field scanning transmission electron microscope (HAADF-STEM) is a powerful method to characterize nanomaterials in 3D at the nanometre scale from a series of 2D electron microscopy images [14] , [15] . Indeed, the contrast in HAADF-STEM images depends monotonically on the sample thickness, which is consistent with tomography criteria for the reconstruction and shows some chemical sensitivity [16] . This makes it ideal to study materials with very different average atomic numbers. Thereby, electron tomography is quite widely used to study the nanoparticle distribution on their support in different catalyst materials [17] and particularly in fuel cell electrodes [18] , [19] , [20] , [21] . In the case of MEAs, the Nafion ionomer consists of a polytetrafluoroethylene (Teflon) backbone with perfluorovinyl ether chains terminated by sulfonate groups as side chains. This ionomer does not present sufficient electronic contrast as compared with the CB to be properly imaged in a HAADF-STEM mode. However, the electron density contrast can be dramatically enhanced by selectively staining the ionic domains with Cs + ions [22] . For this purpose, we studied a model active layer that is prepared with an ink consisting of CB instead of CB supporting Pt nanoparticles in order to avoid perturbing the STEM images with the high-contrast Pt nanoparticles [21] . The ionomer was stained with Cs + ions after coating the ink on the gas diffusion layer using the usual method as for processing an electrode. Two samples were prepared from inks with different compositions: ink for sample 1 has 33 wt% content of Nafion (Nafion/CB=0.5 w/w), which is the widely used content in the electrode of PEMFCs, whereas sample 2 was prepared from an ink containing nearly twice as less Nafion, that is, 17 wt% (Nafion/CB=0.2 w/w). 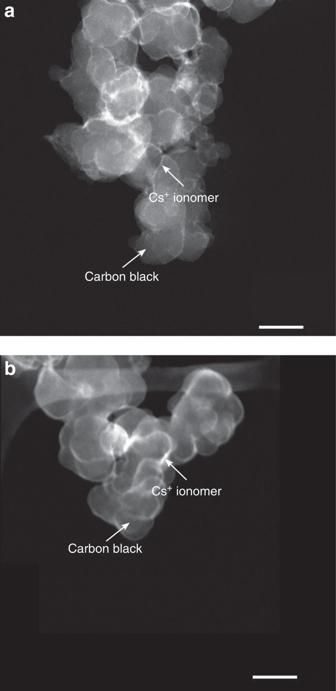Figure 1: 2D imaging of the Nafion/CB nanocomposites in the electrodes of PEMFCs. (a) HAADF-STEM representative micrograph of sample 1 with composition Nafion/CB=0.5 w/w. As the intensity of the HAADF-STEM signal is roughly proportional toZ2, the highest intensities thus correspond to the presence of the Cs+ionomer (ZCs=55), whereas the darker regions are attributed to the CB support (ZCB=6). (b) Same for sample 2 with composition Nafion/CB=0.2 w/w. The scale bars correspond to 100 nm. Figure 1 shows a representative HAADF-STEM image of Cs + -stained sample 1 ( Fig. 1a ) and sample 2 ( Fig. 1b ) extracted from a tomography series taken at different tilt angles. Bright areas surrounding darker agglomerated regions are clearly observed in the micrographs that correspond to the Nafion layer. Such images can provide an estimate of the thickness of the ionomer layer but not a full picture of its distribution because of the 3D structure of the sample, thus not providing any information regarding the degree of coverage of the CB by the ionomer. The present work shows that the combination of HAADF-STEM tomography with the most advanced tomographic reconstruction algorithm can (i) provide a full 3D view of such structure and (ii) by tomogram analysis allows to extract relevant quantitative information. Figure 1: 2D imaging of the Nafion/CB nanocomposites in the electrodes of PEMFCs. ( a ) HAADF-STEM representative micrograph of sample 1 with composition Nafion/CB=0.5 w/w. As the intensity of the HAADF-STEM signal is roughly proportional to Z 2 , the highest intensities thus correspond to the presence of the Cs + ionomer ( Z Cs =55), whereas the darker regions are attributed to the CB support ( Z CB =6). ( b ) Same for sample 2 with composition Nafion/CB=0.2 w/w. The scale bars correspond to 100 nm. Full size image To reconstruct the 3D structure, we used an algorithm based on compressed sensing [23] . The main advantage of this algorithm is to minimize artefacts such as the false elongation resulting from the ‘missing wedge’, thus providing a higher accuracy of reconstruction even with a low number of projections (see Supplementary Methods and Supplementary Fig. 1 for more details). Orthoslices for samples 1 and 2 are displayed in Fig. 2a,b , respectively. As one can notice, the Nafion layer can be clearly observed on the supporting CB particles in the orthoslices. 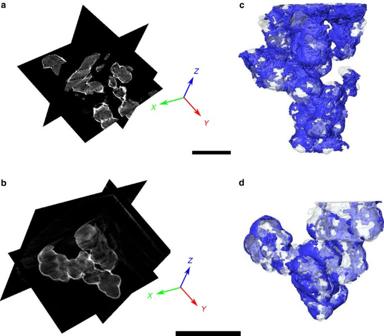Figure 2: Electron tomography imaging of the Nafion layer deposited on CB in the electrodes of PEMFCs. After reconstructing the volume, orthoslices corresponding to one slice of the tomogram can be extracted in planes of whatever orientation as compared with the direction. (a,b) Three representative orthoslices parallel or perpendicular to the incident electron beam axis (along thezdirection) extracted from the reconstructed tomograms for sample 1 (Nafion/CB=0.5 w/w) and sample 2 (Nafion/CB=0.2 w/w), respectively. (c) 3D-rendered volume of sample 1 obtained by segmentation of the HAADF-STEM-reconstructed tomogram. The blue and grey regions correspond to the Cs+-stained ionomer and to the CB support, respectively. (d) Same for sample 2. The scale bars correspond to 200 nm. Figure 2: Electron tomography imaging of the Nafion layer deposited on CB in the electrodes of PEMFCs. After reconstructing the volume, orthoslices corresponding to one slice of the tomogram can be extracted in planes of whatever orientation as compared with the direction. ( a , b ) Three representative orthoslices parallel or perpendicular to the incident electron beam axis (along the z direction) extracted from the reconstructed tomograms for sample 1 (Nafion/CB=0.5 w/w) and sample 2 (Nafion/CB=0.2 w/w), respectively. ( c ) 3D-rendered volume of sample 1 obtained by segmentation of the HAADF-STEM-reconstructed tomogram. The blue and grey regions correspond to the Cs + -stained ionomer and to the CB support, respectively. ( d ) Same for sample 2. The scale bars correspond to 200 nm. Full size image A carefully controlled binarization process was performed to separate the ionomer voxels from the CB ones in order to segment the tomograms and extract the most relevant morphological parameters of the Nafion layer ( Fig. 3 and Supplementary Fig. 2 ). The 3D distribution of the Nafion layer on the CB is highlighted in the surface-rendered tomograms for samples 1 ( Fig. 2c ) and 2 ( Fig. 2d ): the Cs + ionomer is represented in blue and the CB support in transparent grey (see Supplementary Movie 1 and Supplementary Movie 2 for 3D view of sample 1 and sample 2, respectively). Qualitatively, a nonuniform distribution of the ionomer layer is revealed for both samples and a larger fraction of area of the CB appears to be coated by the ionomer in sample 1 as compared with sample 2. To gain further insight into the differences in the coated area between the two samples, a quantification of the binarized tomograms was performed. 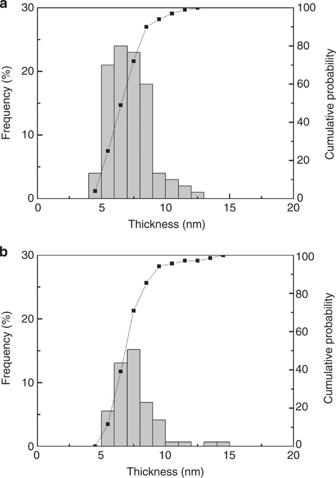Figure 3: Thickness of the Nafion layer. (a) Distribution of the thickness of the Nafion layer deposited on CB for sample 1 (Nafion/CB=0.5 w/w). The histogram is derived from ~100 measurements performed in different zones of the reconstructed tomogram. The black dotted curve corresponds to the cumulative distribution of the ionomer layer thickness. (b) Same for sample 2 (Nafion/CB=0.2 w/w). Figure 3: Thickness of the Nafion layer. ( a ) Distribution of the thickness of the Nafion layer deposited on CB for sample 1 (Nafion/CB=0.5 w/w). The histogram is derived from ~100 measurements performed in different zones of the reconstructed tomogram. The black dotted curve corresponds to the cumulative distribution of the ionomer layer thickness. ( b ) Same for sample 2 (Nafion/CB=0.2 w/w). Full size image Ionomer layer morphological feature from electron tomogram Important parameters that can be extracted from the segmented volume are the volume fraction, the degree of coverage and the average thickness of the ionomer layer ( Table 1 ). The measured volume fraction of Nafion in sample 1 is around two times larger than that for sample 2 as expected from the ink composition. However, the total ionomer volume fraction measured on the two samples is smaller than the expected one: 20 and 13% instead of 33 and 17% for samples 1 and 2, respectively. One possible explanation to this discrepancy is that a significant fraction of the Nafion present in the ink agglomerates to form ionomer ‘pockets’ in the electrodes, as was observed by More et al. [12] The formation of these Nafion pockets might be a direct consequence of the broad distribution of ionomer particle sizes ranging up to micrometre large aggregates in the Nafion dispersions [24] . Thus, our present results indicate that for sample 1 only ~60% (and 76% for sample 2) of the ionomer present in the ink is available for covering uniformly the CB particles. Table 1 Quantified morphological data extracted from the binarized reconstructed volumes obtained with HAADF-STEM electron tomography. Full size table Other important parameters as the average thickness of the ionomer and the degree of coverage ( δ ) of the CB nanoparticles have also been quantified ( Table 1 ). These parameters are known to have a high impact on the performance of the fuel cells as they play a crucial role in the transport processes of protons and gaseous reactants. The thickness of the ionomer layer was quantified by a statistical analysis of the particle edges in the tomograms ( Supplementary Fig. 4 ). The histograms, displayed in Fig. 3 , are very close for the two samples: the average thickness amounts to 7.2 and 7.6 nm for samples 1 and 2, respectively, with ~95% of the measured thicknesses being within the range of 4.5–9.5 nm in both cases. Such values are not only in good agreement with those previously reported in the literature [12] , [13] but are also consistent with the ability of Nafion to form thin films and to coat evenly any media whether hydrophilic or hydrophobic [25] , [26] , [27] , [28] . Such a property has been recently confirmed through the fabrication and characterization of physical–chemical properties of Nafion films with a thickness of several nanometres [29] , [30] . Moreover, the thickness of the layer derived from the present study corresponds to the smallest characteristic dimension of polymer aggregates in Nafion dispersions [31] . In suspensions, Nafion forms elongated aggregates similar to that of ribbons with a rectangular cross-section of ~3 by 10 nm as was evidenced by small angle X-ray and neutron scattering [31] . This means that the shape of these aggregates does not change significantly upon processing the ink and they are deposited homogeneously on the CB particles until their entire surface is covered. In the present work, the ionomer distribution analysis was purposely performed using an ink consisting of CB without Pt nanoparticles as these would give a too high contrast in the tomograms as compared with the Nafion layer and the CB particles. We thus performed high-resolution TEM additional analysis on a scratched real catalyst layer ( Supplementary Fig. 5 ). Although the Nafion layer is not always easily observed in high-resolution TEM mode, the presence of Pt nanoparticles does not appear to affect the coverage of the CB nanoparticles by the Nafion layer; on these images, the Nafion layer thickness is in the same range as the one measured when performing tomography on the model system ( Fig. 2 ). On the other hand, the tomography analysis clearly shows a large difference between the two samples in terms of the covered area δ (in %) of the supporting CB nanoparticles: whereas it amounts to 79.5±2.3% for sample 1, it is only 49.9±1.2% for sample 2 ( Table 1 ). Therefore, dividing the amount of ionomer by a factor of two in the processing ink does not influence the thickness of the layer of ionomer but rather leads to a lower coverage of the CB nanoparticles. These quantitative data provided by electron tomography on the Nafion thin layer can be directly related to the variations of the electrochemical performance of the related electrode and of the derived fuel cell with the amount of ionomer in the processing ink. It is indeed reported that the optimal Nafion content in the catalytic ink is 30±6% wt% [32] . Lee et al. [10] , through measurements of the electrochemically active surface area (number of Pt nanoparticles in contact with the ionomer electrolyte), showed that the connectivity of the proton conduction paths is improved when the Nafion content increases from 23 to 40%. They explained their results by a larger number of Nafion-coated Pt nanoparticles, while the polymer film thickness remains constant. This is in agreement with our present 3D analysis. We therefore propose the following scenario: (i) for a low Nafion content, the CB grains are partially covered by Nafion; thus, only a reduced percentage of Pt nanoparticles will be in contact with the ionomer, providing poor connectivity and therefore inducing a higher resistance to the proton flow into the active layer towards the membrane. (ii) For the optimal Nafion content, nearly all CBs are covered by Nafion, thus leading to a larger electrochemically active area. The thickness layer remains constant, around 7 nm, and does not restrain O 2 diffusion. Eventually, (iii) a further increase in the Nafion content leads to a thicker ionomer layer, which then becomes a significant O 2 diffusion barrier leading to deteriorated performances. To conclude, HAADF-STEM electron tomography was successfully used to image Nafion ultrathin layers in the electrodes of PEMFCs. This is the first experimental study of the Nafion layer in fuel cell electrodes providing quantitative morphological parameters (average thickness, degree of coverage of the CB-supporting particles). These results allow a direct correlation of the 3D Nafion layer structure to the electrochemical response of the electrode. This accurate 3D analysis is of great interest for describing the electrode microstructure, such description being needed for electrochemical models aiming at predicting the performance of a fuel cell. An extension of the present work will be carried out to study the impact on the ionomer layer structure, and hence on the electrode properties, using different types of ionomer as well as other ink or electrode-manufacturing processes. In addition, the present methodology based on nanoscale tomography analysis should be of interest for many other problems where the surface coverage and the 3D structure of nano-objects and nanomaterials by a thin nanometre-thick layer is involved such as in nanocomposite material batteries, third-generation organic and hybrid solar cells or new catalysts for environmental catalysis. Sample preparation Slurries have been prepared by mixing CB nanoparticles Vulcan XC72 from Cabot with commercial suspension of Nafion D2020 from Dupont (20 wt% in water and isopropanol mixture of ionomer with an equivalent weight of 1,000 g eq −1 ) into a mixture of pure ethanol and ultrapure water. The dry content was 23 wt%. Samples have been fabricated by coating the slurries on a commercial Gas Diffusion Layer SGL24BC from SGL Carbon. Two samples have been prepared with 17 and 33 wt% of Nafion in the ink. To perform the tomographical HAADF-STEM analysis of the Nafion deposited on CB nanoparticles, a small part of the GDL coating was scratched and dispersed in a saturated solution of Cs 2 SO 4 in water during 72 h in order to exchange the sulfonic acid sites by Cs + . We used Cs + cations rather than uranyl UO 2 2+ ones because their monovalent character allows a double loading as compared with divalent cations. Floating particles of CB were then transferred on lacey carbon-coated Cu TEM grids (Agar Ref: S166-3). Electron tomography HAADF-STEM electron tomography was carried out on a LB FEI TITAN 80-300 electron microscope equipped with a probe C s corrector operating at 200 kV and using a Fischione 2020 single-tilt tomography holder. Before recording a series of images, aberrations of the condenser lenses were corrected up to second order using the Zemlin tableau. A convergence angle of 10 mrad and 128 mm of camera length were used. Using the ‘3D Explorer’ FEI software, the data collections were performed by tilting the specimen around a single axis perpendicular to the electron beam between −76° and +72° for Cs + -ionomer-1, and between −72° and +66° for Cs + -ionomer-2 and using 2° steps. The range of achievable tilting angles is limited by the shadowing effect of the grid when using too large angles. In order to reconstruct tomograms, the registered tilt series were aligned using the FEI Inspect 3D software and a software written in MATLAB. In particular, compressed sensing algorithm was applied as described in the Supplementary Information . The reconstructed volumes were thereafter processed using the Avizo 6.0 Fire edition and the Fiji software, further details being provided in the Supplementary Information . How to cite this article: Lopez-Haro, M. et al. Three-dimensional analysis of Nafion layers in fuel cell electrodes. Nat. Commun. 5:5229 doi: 10.1038/ncomms6229 (2014).